Level statistics of disordered spin-1/2 systems and materials with localized Cooper pairs The origin of continuous energy spectra in large disordered interacting quantum systems is one of the key unsolved problems in quantum physics. Although small quantum systems with discrete energy levels are noiseless and stay coherent forever in the absence of any coupling to external world, most large-scale quantum systems are able to produce a thermal bath and excitation decay. This intrinsic decoherence is manifested by a broadening of energy levels, which aquire a finite width. The important question is: what is the driving force and the mechanism of transition(s) between these two types of many-body systems - with and without intrinsic decoherence? Here we address this question via the numerical study of energy-level statistics of a system of interacting spin-1/2 with random transverse fields. We present the first evidence for a well-defined quantum phase transition between domains of discrete and continous many-body spectra in such spin models, implying the appearance of novel insulating phases in the vicinity of the superconductor–insulator transition in InO x and similar materials. Although quantum phase transitions between regimes with and without intrinsic decoherence were first discussed by Anderson in 1958 (ref. 1 ), their understanding is still incomplete. More recently, a number of works have studied these transitions in strongly disordered electron systems with weak repulsion [2] , [3] , [4] and reached the conclusion [3] , [4] that a finite-temperature phase transition takes place between two regimes, 'weakly insulating' and 'strongly insulating', that are characterized by non-zero and zero linear conductivities, respectively. In terms of the many-particle excitation spectra, this result translates into the existence of an extensive (proportional to the volume of the system) energy threshold, with a critical excitation energy ɛ c ∝ υT c that separates the discrete spectrum of excitations at E < ɛ c and continous one at E > ɛ c for any large but finite subsystem of size υ . It also implies that the low-temperature state is free from decoherence because the lifetime of all excitations is infinite. The phase transition predicted in ref. 4 would imply that the resistivity of the material shows a faster-than-activated growth when the temperature is decreased. In contrast, in ordinary hopping insulators, one usually observes that the conductivity vanishes continously at T →0: , with a <1, that is, slower than activated. Some of the best systems to test general theoretical ideas [4] are the insulators formed by adding disorder to a class of superconductors that do not lose their pairing gap upon the introduction of disorder. Different physical properties of the excitations at low and high energies in the infinite system are reflected in different statististical properties of the spectra of finite systems at E<ɛ c and at E>ɛ c . Intuitively, if the eigenvectors are extended, as expected for the state where local excitations decay, they are subject to inter-level repulsion. Conversely, if the eigenvectors are localized, eigenvalues corresponding to excitations localized in different parts of the system are independent and one expects a Poisson distribution of energy levels. The amount of disorder can be characterized by an interaction constant g (which decreases when the disorder increases). At some value g c of this interaction constant, the low energy excitations get localized. Exactly at g=g c , only the lowest energy excitations are localized. When one increases the disorder further, the low-energy excitations, with energy ω<ɛ c ( g ), are localized, whereas all higher-energy excitations remain delocalized. In this regime, the threshold energy ɛ c is intensive [5] , [6] (it does not grow with the size of the system), so that the density of mobile excitations is proportional to exp(− ɛ c / T ), leading to the activated behaviour of all transport quantites. A similar picture was proposed in ref. 7 on the basis of phenomenological arguments but criticized in ref. 8 and reconsidered in ref. 9 . At even stronger disorder, g = g *, the threshold energy ɛ c ( g ) diverges. In the opposite limit of large g (low disorder), one expects the formation of long-range order. In the model studied analytically in refs 5 , 6 and its generalization studied here, the long-range order is formed at the same point g c at which the lowest energy states become delocalized. The divergence of the threshold ɛ c at g→g * might be cut-off by the system size, so that at stronger disorder ɛ c scales with the system volume, υ . In this case, one gets the finite temperature transition between weak and strong insulators predicted in refs 3 , 4 . However, it is also possible that the energy scale ɛ c becomes really infinite at g → g *, which implies, for g < g *, a complete localization and the absence of a thermal equilibrium at all temperatures. The goal of the present paper is to provide a qualitative picture of the many-body localization for a system of interacting spins-1/2 in a site-random transverse field using a direct numerical study. These computations take into account the whole excitation spectrum. We will give evidence that both situations mentioned above (with and without temperature-driven transition) can be realized in discrete spin models, depending on the detailed form of the Hamiltonian. The model that we study below captures the main ingredients of the physics of the superconductor–insulator transition in amorphous disordered superconductors, InO x and TiN x , and the predictions of the theory are in agreement with the data on these materials. The Hamiltonian and general phase diagram The simplest and most physical model that describes the disorder-driven formation of insulating phases in the many-body systems described above is the spin model where points i,j belong to a random graph G with a fixed coordination number are spin-1/2 operators, , the sum goes over all different pairs of nearest neighbours i,j on G , and all non-zero matrix elements are equal to . The random values ξ j are uncorrelated at different sites and chosen from the box distribution , corresponding to a bandwidth equal to W in terms of local energies . The model has three ingredients: random fields ξ i in z directions that form localized levels, a J xy coupling that tries to delocalize the spin excitations and lead to an ordered state at large J xy , and a J zz coupling that is essential for the temperature-driven transition between weak and strong insulators. The general phase diagram that describes different many-body states corresponding to the Hamiltonian (1) is shown in Fig. 1 ; it summarizes the results of the present study. In the models without s z s z interaction, we find that ɛ c is infinite at g < g *, but the presence of this interaction results in the appearance of a narrow range g I < g < g* where ɛ c is extensive, signalling the existence of a finite-temperature transition in this regime even for a small interaction constant J zz . 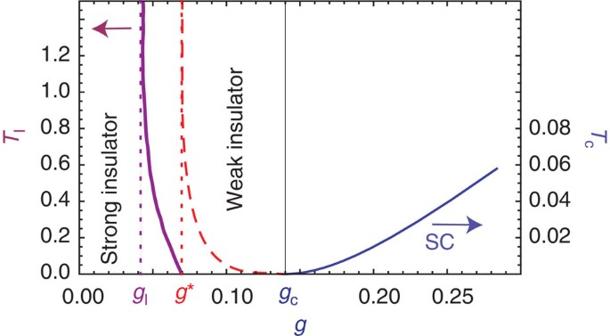Figure 1: Phase diagram in the temperature-coupling constant plane. The phase diagram is obtained from the solution of cavity equations for the model (1) withZ=K+1=3 and confirmed by numerical simulations. Blue line shows the dependence of the critical ordering temperatureTc(g) on the coupling constant atg>gc. The strength of theszszinteraction isJzz=0.4, non-zeroJzzresults in ag-dependent line (purple) separating weak and strong insulators; in the absence ofszszinteraction, this line becomes vertical. In the weak insulator, excitations at sufficiently high energies can decay even at zero temperature (the corresponding energy threshold is shown forJzz=0 by the dashed red line). A non-zero temperature results in non-zero relaxation of all excitations, even the ones of lowest energy. In contrast, in the strong insulator, no excitation with intensive energy can decay. As the interaction constantgis decreased, the temperature separating these phases (purple line) goes to infinity atg=gI. At smaller couplingg<gI, all excitations, even those with extensive energy, remain localized. The value ofgI≈0.042 is approximately equal to 0.30gc. The ratiogI/gc=0.3 is in good agreement with the results of the direct diagonalization on small graphs, as can be seen from the critical values offound inFig. 4: 0.022 for the middle of the band and 0.081 for the low energies. Figure 1: Phase diagram in the temperature-coupling constant plane. The phase diagram is obtained from the solution of cavity equations for the model (1) with Z = K +1=3 and confirmed by numerical simulations. Blue line shows the dependence of the critical ordering temperature T c ( g ) on the coupling constant at g > g c . The strength of the s z s z interaction is J zz =0.4, non-zero J zz results in a g -dependent line (purple) separating weak and strong insulators; in the absence of s z s z interaction, this line becomes vertical. In the weak insulator, excitations at sufficiently high energies can decay even at zero temperature (the corresponding energy threshold is shown for J zz =0 by the dashed red line). A non-zero temperature results in non-zero relaxation of all excitations, even the ones of lowest energy. In contrast, in the strong insulator, no excitation with intensive energy can decay. As the interaction constant g is decreased, the temperature separating these phases (purple line) goes to infinity at g = g I . At smaller coupling g < g I , all excitations, even those with extensive energy, remain localized. The value of g I ≈0.042 is approximately equal to 0.30 g c . The ratio g I / g c =0.3 is in good agreement with the results of the direct diagonalization on small graphs, as can be seen from the critical values of found in Fig. 4 : 0.022 for the middle of the band and 0.081 for the low energies. Full size image The phase diagram shown in Fig. 1 has another important feature: it predicts a direct transition between the ordered state and the insulator, with characteristic energy scales that go down to zero continously on both sides of the transition. In the ordered state, this energy scale is given by the typical value of the order parameter or the transition temperature, whereas in the insulating states it is the value of the threshold energy ɛ c ( g ), which implies the Arrhenius behaviour of the resistivity at very low temperatures. Below we present the derivation of this phase diagram as well as other results of our study. Level statistics and quantum phase transition The eigenstates of the Hamiltonian (1) are vectors in the 2 N -dimensional Fock space ( N is the total number of sites of G ). As discussed in the introduction, the transition between decoherent and coherent states can be deduced from the change in the statistics of the exact eigenvalues E i of the Hamitlonian. These arguments can be made more rigorous by noting that the statistical properties of the spectra on one hand, and the possibility of energy transport on the other hand, are both related to the response to the 'gravitational' potential [10] that modifies the Hamiltonian by where φ ( t , x ) is a generic slow function of coordinates and time. A small perturbation of this type results in a slow (adiabatic) motion of the energy levels E n ( t ). In the absence of level repulsion, different levels cross without affecting each other, so that this motion only affects the total phase of the wave function. Because the field is conjugated to the energy density, the absence of response to it implies the absence of energy transport (and therefore a zero thermal conductivity). An excitation with energy Δ E localized around point x acquires a phase due to the perturbation (2); in contrast, a delocalized excitation becomes a superposition of other excitations. Thus, the absence of a response also implies that excitations are localized and do not decay. We conclude that (in a generic quantum system) the absence of level repulsion implies the spatial localization of excitations, the absence of their decay and of the thermal current, that is, the formation of a strong insulator. Because level statistics can be studied for relatively small systems, this correspondence between the level statistics and the physical properties in the thermodynamic limit provides a convenient numerical tool to predict the properties of physical systems. This strategy has been used for instance in ref. 11 for the study of interacting fermionic system. To characterize the statistics of energy levels, we study the dimensionless parameter r n ∈ [0,1] defined as where δ n = E n − E n −1 and E n is the n -th energy level. The average value r =〈 r n 〉 is equal to 0.38 for Poisson level statistics, and to 0.53 for Wigner–Dyson statistics. In the limit of infinite systems, one expects a sharp transition between these two values as a function of g , or of the energy. In a finite system, the parameter r increases smoothly, but the curve r ( g ) is expected to become steeper as the size is increased. The appearance of a unique crossing point of these curves for different sizes N implies a well-defined phase transition in the limit of infinite-size systems. Such a crossing point is clearly seen in the exact diagonalization of the Hamiltonian (1) with Z =3, shown in Fig. 2 for J zz =0. Apart from the persistance of the transition for small system sizes, these data also show that the critical value of J xy changes very little, as the energy is increased to the centre of the band. This proves that high-energy states in this model become localized together with the low-energy ones, in more physical terms, it implies that no new decay channels appear at high energies. The absence of new decay processes at high energies is the physical reason why one does not find an intermediate phase with extensive energy threshold in this model. Also, these data show that the transition happens at a value r n ( g ) that is close to its value 0.38 expected for Poisson statistics. This is due to a large distribution of relaxation rates in these systems [6] , which implies that in case of small systems, many realizations of the random energies give localized states, while delocalization only happens with a small probability, as we explain in more detail below. Finally, the critical value of J xy coincides with the prediction of the analytical theory adjusted for the systems of these sizes as shown in Fig. 3 ; in this theory, the main effect of the finite system size is the appearance of a bimodal distribution function that corresponds to a finite probability to find a sample with zero level width; this effect shifts the critical value g upwards (see Methods). 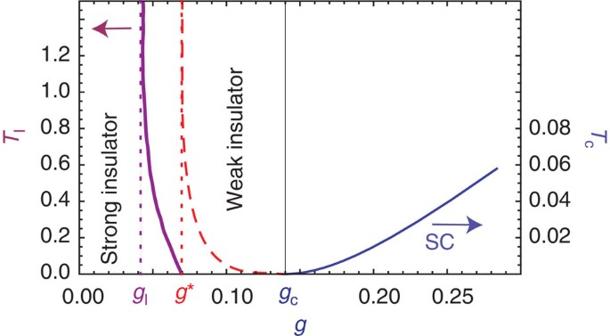Figure 2: Evolution of the energy level statistics. The average parameter 〈rn〉 that distinguishes Wigner–Dyson and Poisson distributions (values of 〈rn〉 corresponding to these distributions are shown by horizontal dashed lines) is plotted versus the transverse interaction constant,Jxy. The numerical study refers to the sector withfor the model (1) withJzz=0, defined on aZ=3 random graph with bandwidthW=1. Panelashows the statistics of the low-energy excitations in the energy interval (Egs,Egs+1.5). Data points are shown for system sizesN=14 (black dots),N=16 (red),N=18(blue),N=20 (green) andN=22 (violet). The critical value of the couplingis determined via a crossing point analysis. Panelbshows similar results for intermediate excitation energies, (Egs+1.5,Egs+2.5), leading to the critical point. Panelccorresponds to high energies, close to the centre of the many-body spectrum, with the critical point. Each data point represents the average overNr=2,000, 200, 100 and 60 disorder realizations forNS=14, 16, 18 and 20, respectively. A large (exponential) increase in the number of states implies that larger samples require less averaging over realization to achieve the same accuracy. Figure 2: Evolution of the energy level statistics. The average parameter 〈 r n 〉 that distinguishes Wigner–Dyson and Poisson distributions (values of 〈 r n 〉 corresponding to these distributions are shown by horizontal dashed lines) is plotted versus the transverse interaction constant, J xy . The numerical study refers to the sector with for the model (1) with J zz =0, defined on a Z =3 random graph with bandwidth W =1. Panel a shows the statistics of the low-energy excitations in the energy interval ( E gs , E gs +1.5). Data points are shown for system sizes N =14 (black dots), N =16 (red), N = 18 (blue), N =20 (green) and N =22 (violet). The critical value of the coupling is determined via a crossing point analysis. Panel b shows similar results for intermediate excitation energies, ( E gs +1.5, E gs +2.5), leading to the critical point . Panel c corresponds to high energies, close to the centre of the many-body spectrum, with the critical point . Each data point represents the average over N r =2,000, 200, 100 and 60 disorder realizations for N S =14, 16, 18 and 20, respectively. A large (exponential) increase in the number of states implies that larger samples require less averaging over realization to achieve the same accuracy. 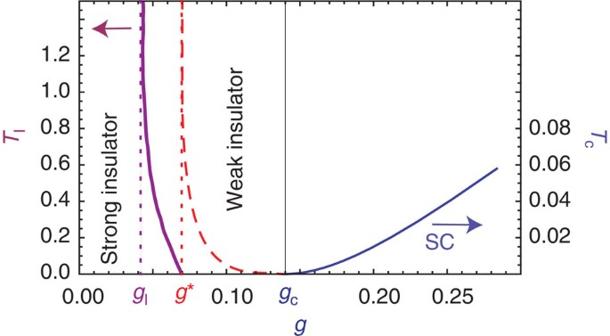Figure 3: Phase diagram and finite-size effects. Phase diagram for the model (1) withJzz=0 as a function of the interaction constantg. The full lines show the predictions of the analytical study of the model (1) for the critical temperature (right vertical axis) and the threshold energy,ɛ, (left axis) of spin-flip excitations in infinite random graphs withZ=3 neighbours. The vertical ovals show the values of the critical coupling constant that correspond to a transition between different types of spectra for different energiesEin finite random graphs of small size (N=16–20) as determined by direct numerical simulations. The uppermost oval shows the transition at the many-body band centre (corresponding toE≫1) that sets a lower bound for the criticalg(E). The thick dashed line shows the position of the spectral threshold for single-spin excitations with energyɛadjusted by finite-size effects, as explained in the main text and in the Methods section. The small circles show the typical energy of the single-spin excitations,ɛ(E), that gives the main contribution to the many body excitations studied in direct numerical simulations. The good agreement between their position and expectations (dashed line) confirms the validity of the cavity method5,6that is used to obtain the results in infinite systems. The very small change in the critical value of the coupling constant between excitations at energyE≈2.0 and the centre of the many-body band implies that all excitations, at high and low energies, become localized wheng<g*. Full size image Figure 3: Phase diagram and finite-size effects. Phase diagram for the model (1) with J zz =0 as a function of the interaction constant g . The full lines show the predictions of the analytical study of the model (1) for the critical temperature (right vertical axis) and the threshold energy, ɛ , (left axis) of spin-flip excitations in infinite random graphs with Z= 3 neighbours. The vertical ovals show the values of the critical coupling constant that correspond to a transition between different types of spectra for different energies E in finite random graphs of small size ( N= 16–20) as determined by direct numerical simulations. The uppermost oval shows the transition at the many-body band centre (corresponding to E ≫ 1) that sets a lower bound for the critical g ( E ). The thick dashed line shows the position of the spectral threshold for single-spin excitations with energy ɛ adjusted by finite-size effects, as explained in the main text and in the Methods section. The small circles show the typical energy of the single-spin excitations, ɛ ( E ), that gives the main contribution to the many body excitations studied in direct numerical simulations. The good agreement between their position and expectations (dashed line) confirms the validity of the cavity method [5] , [6] that is used to obtain the results in infinite systems. The very small change in the critical value of the coupling constant between excitations at energy E ≈2.0 and the centre of the many-body band implies that all excitations, at high and low energies, become localized when g < g *. Full size image The agreement between the results of the cavity approximation [5] , [6] and that of the numerical diagonalization of small random graphs implies that small loops appearing in random graphs are irrelevant for the formation of the coherent states. This is not unexpected because the decoherence in this model is associated with the spin-flip processes that couple rare pairs of spins that are almost in resonance with each other. These pairs form a very dilute network without loops. This conclusion implies that the cavity approximation provides a very good starting point for the description of the realistic system as well. S z – S z coupling and finite- T phase transition We now argue that the absence of an intermediate phase with extensive energy threshold found in the study above was due to the absence of interactions between individual spin flips ( J zz =0). At non-zero J zz , the first two terms in the Hamiltonian (1) describe a classical Ising magnet in a random field. We shall be interested in its disordered phase, which is realized when the longitudinal interaction is small, J zz < W . In this case, the classical eigenstates of this magnet coincide with those of independent spins, with energies that are weakly modified by the interaction. In the absence of transverse interactions, the excitations of this magnet are individual spin flips with energies . In the ground state, the direction of almost all spins is determined by the sign of the random field, so the presence of a small J zz affects weakly the density of states of these low-energy excitations and their decay due to transverse interactions. Thus, we expect that the low-energy properties of the spectrum remain similar to the model with zero J zz . The situation is very different at high energies when the decay of a given spin occurs against the background of different spin configurations. Physically, a spin excitation at energy ɛ has a much larger chance to propagate through a given site if the energy of the spin flip at this site is close to ɛ . The energy of a spin flip is distributed with the probability density Q (ξ), where ξ= ɛ / W , if all surrounding spins are locked into a fixed configuration. In contrast, at extensive energies (corresponding to non-zero temperatures), the surrounding spins acquire many different configurations. This increases the probability that a given site is in resonance with the excitation. This effect can be also described as being due to the interaction between individual spin-flip processes that allow new channels for the decay of these excitations. This should result in the large suppression of the critical value of the interaction constant at high energies. This effect is not sensitive to the sign of J z < W . The exact diagonalization of the Hamiltonian on a Z =3 random graph with J zz =0.4 confirms these expectations ( Fig. 4 ). Non-zero value of J zz decreases slightly the value of g c at low energies ( J c =0.095→0.081). This decrease becomes substantial for medium energies ( J c =0.066→0.044) and very large for energies close to the band centre: J c =0.061→0.022. A slight and moderate decrease of the critical value of the interaction constant at low and medium energies is probably due to the fact that at these energies a typical excited state contains more than one spin-flip excitation. As explained above, the interaction between these excitations leads to delocalization. 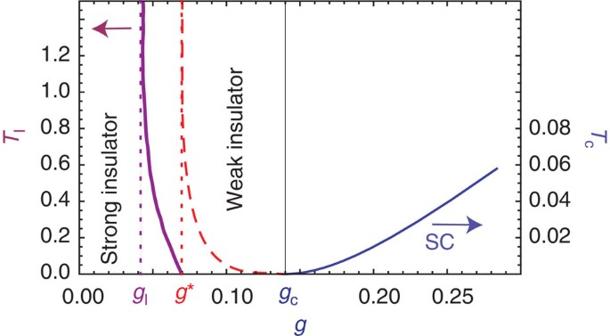Figure 4: Level statistics in presence of longitudinal spin coupling. The evolution of the average parameter 〈rn〉 as a function ofJxyis studied for thesector of the model (1) withJzz=0.4, defined on aZ=3 random graph with bandwidthW=1. Data forN=16, 18, 20 spins are represented by red, blue and green points, respectively. Panelashows data for low excitation energiesE≤1.5, leading to the critical point at; in panelb, the data for the intermediate energy intervalE∈(1.5, 2.5) are shown, with; finally, panelccorresponds to the centre of the many body band, where. Panelsbandcdemonstrate (compare withFig. 2b and c) a large effect due to a small longitudinal couplingJzz=0.4: it shifts the crossing point to much smaller values of the transverse couplinggfor high-energy states. Figure 4: Level statistics in presence of longitudinal spin coupling. The evolution of the average parameter 〈 r n 〉 as a function of J xy is studied for the sector of the model (1) with J zz =0.4, defined on a Z =3 random graph with bandwidth W =1. Data for N =16, 18, 20 spins are represented by red, blue and green points, respectively. Panel a shows data for low excitation energies E ≤1.5, leading to the critical point at ; in panel b , the data for the intermediate energy interval E ∈ (1.5, 2.5) are shown, with ; finally, panel c corresponds to the centre of the many body band, where . Panels b and c demonstrate (compare with Fig. 2b and c ) a large effect due to a small longitudinal coupling J zz =0.4: it shifts the crossing point to much smaller values of the transverse coupling g for high-energy states. Full size image The solution of the cavity equations, similar to those solved in ref. 6 (see below) confirms the appearance of the extensive threshold for J zz ≠0 and gives the dependence of the transition temperature T I ( g ) on the coupling constant g that we show in Fig. 1 for J zz =0.4. At g < g * and T < T I ( g ), all excitations with intensive energies are localized, no transport of any sort is possible. In contrast, at higher temperatures T > T I ( g ) all excitations, even those with low energies, acquire a non-zero width. At g > g* and zero temperature, the excitations with low energy are localized, whereas high-energy excitations decay. This distinction is smeared at any non-zero temperature because the presence of even a small density of mobile high-energy excitations leads to a slow decay of even the lowest-energy ones. In the previous papers [5] , [6] , we derived a recursion relation for the intrinsic level widths of single-spin-flip excitations, assuming a local Bethe lattice structure of the lattice: where k ( i ) are the K =Z−1 neighbours of i in the cavity graph. The same recursions can be used for a random graph model studied in the present paper, upon neglecting the contributions of closed loops (loops are totally absent on the infinite Bethe lattice, whereas they are present with parametrically low density ∼ 1/ln N on a random graph with N sites). The condition of stationarity of the distribution function generated by the mapping (4) leads to the solution for typical found in ref. 6 . In presence of coupling, the recursion equation (4) should be modified. At non-zero temperature T = β −1 it contains the sum over neigboring spin configurations with their thermal weights: where the internal summation over includes all configurations of spin variables connected to the spin s k by z−z links, are the corresponding local partition functions, and The largest contribution to the sum (4) comes from the site k characterized by ξ k that is closest to ω . The same holds for the sum (5), but, in addition, in this sum the value of ɛ k varies depending on the surrounding spins. This increases the probability to find a resonance. To evaluate the importance of this effect, we consider explicitly the case of Z =3 (corresponding to the random graphs diagonalized in this paper) and the energy at the centre of the band, ω = W /2. The critical value of the coupling constant is determined by the condition in the limit of the large system size. Here is the relaxation rate induced deep in the centre of the lattice when infinitesimally small couplings are added at the boundary, and . The overbar means the averaging over disorder (that is, over the distribution of ξ). Performing the same steps as in ref. 6 , we average over disorder using the replica method and we get the condition for the critical value of g ( T ): where . The inversion of the numerically obtained function g ( T ) provides the T I ( g ) dependence shown in Fig. 1 by the thick purple line. Applications to superconductor–insulator transitions One of the best experimental systems to test these predictions is provided by strongly disordered superconductors such as InO x in the vicinity of the disorder-induced superconductor–insulator transition [12] ; for recent reviews see ref. 13 and the introduction of the paper [14] . One advantage of these systems is that the transition can be fine tuned by a magnetic field. In their insulating state, these systems demonstrate purely activated behaviour , with a =1 (refs 15 , 16 ). Far in the insulating state [12] this behaviour can be understood in terms of a single electron pseudogap [17] , [18] that results from binding of localized electrons [14] , [19] . However, the persistance of an activated behaviour in the vicinity of the superconductor–insulator transition where one expects the appearance of low-energy Cooper pairs requires another explanation. It is natural to ascribe it to the appearance of the many-body mobility edge ɛ c ( g ) introduced above. The appearance of a range g I < g < g * where ɛ c is extensive raises the possibility that a finite-temperature transition between strong and weak insulators might be observed in InO, TiN or similar films very close to the superconductor–insulator transition. The superconductor–insulator transition can be described by the model (1) provided that a strong pseudogap allows one to reduce the Hilbert space of the full electron problem to the one spanned by 'pseudospin'-1/2 variables , that describe [20] creation–annihilation and counting operators of the localized Cooper pairs. The random field in the model (1) in this case describes random electron energy levels, the J xy interaction accounts for the tunnelling of Cooper pairs and the J zz interaction can be viewed as a density–density interaction that is due to the long-range part of the Coulomb interaction ( J z <0) or to phonon-mediated attraction between electrons ( J z >0) [14] . The assumption of a large pseudogap is borne out by experimental results [17] , [18] . On the theoretical side, its origin lies in the fractal stucture of the wave functions near to the mobility edge of the single electron problem [14] , [19] . It is further supported by direct numerical simulations of electrons with attractive interactions in a random potential [21] and by the experimental observation [18] of the anomalous broadening of the order parameter distribution predicted by the theory. The main conclusion of our work is the existence of two different insulating phases and the prediction of a finite-temperature transition between a weak insulator characterized by an activated transport and a strong one in which no transport occurs. These results are obtained within a lattice spin-1/2 model, which serves as a good approximation to the description of the superconductor–insulator transition in disordered systems characterized by a pseudogap. We believe that it might be possible to observe this transition in insulating films in a close proximity to the superconducting transition. Because of a finite value of the pseudogap in a realistic systems, a temperature-driven transition between weak and strong insulating phases will be seen as a sharp crossover in resistivity curves R ( T ), with a rapid growth of the apparent activation energy d ln R ( T )/ d (1/ T ), as T decreases. Some preliminary experimental evidence for this behaviour in TiN was reported in ref. 22 , it was also observed in InO x (B. Sacépé, personal communication). The methods developed in this work and in some case even the qualitative results might be also applied to many other physical systems, such as the disordered spin 1/2 magnets, in which the transition between different phases can be caused by the application of magnetic field (for example, disordered magnets based on strongly anisotropic material CuB 2 O 4 , see ref. 23 ), or the interacting two-level systems at very low temperatures, such that their interaction with phonons become irrelevant. The formation of the coherent states (strong insulator) in these various situations would be crucial for the creation of the noiseless environment of quantum bits. Finally, formation of the coherent states in a strong or even a weak insulator implies that in this phase the physical system has no natural relaxation mechanism and thus remains highly out of equilibrium for a long time, until other physical effects such as phonons establish the equilibrium, the transport in this phase exhibits many anomalies [24] . Critical scaling analysis To compare quantitatively the results of the direct diagonalization shown in Fig. 2 with the predictions of the theory [6] , we need to take into account the finite size effects. The finite size has two effects. First, it results in small shifts of the crossing points for different pairs of curves. This effect can be taken into account by the scaling analysis developed in ref. 25 , by fitting the data to the equation where L is the maximal distance in the space of many body wave functions: and v is a fitting exponent. In practise, we truncated the series with n max =3, we checked that the results are not sensitive (deviations to n max and to the choice of the scaling function, and that they do not change significantly if the largest value of N is limited to 20 instead of 22. The exact value of the crossing point has also a statistical error due to the finite number of samples that were generated. Combining together the statistical errors and the errors from the scaling analysis, we come with the error estimates shown in Figs 2 and 4 . Finite size effects upon the transition line In a finite system, the crossover from Poisson to Wigner–Dyson statistics is expected to occur when the states become delocalized. Delocalization implies that the width of the level , determined self consistently in the cavity approach [6] , is of the order of the level spacing δ ( E )=1/ v ( E ), where the full density of states v ( E ) is an exponential function of the excitation energy, , see Supplementary Methods for the analitic derivation of this dependence (originally found in ref. 26 ), comparison with direct computation of the density of states in the Supplementary Fig. S1 , and with simulation for the simplified model at finite N in the Supplementary Fig. S2 . A number of finite-size effects makes the direct comparison between the analytical results for infinite systems [6] and numerical results reported here non-trivial. First, the width, , of the level is expected to become exponentially small as the energy threshold is approached: Furthermore, the coefficient, ω 1 , in this equation is much larger (see ref. 6 ) than ɛ c , so the decay rate becomes very small even relatively far from the transition line. In a finite system with a not-so-small level spacing, this leads to a very significant shift of the apparent critical energy due to finite-size effects. Second, the width of the levels fluctuates strongly from one graph realization to another, see inset in Fig. 5 . The large peak at small values of shows that in many realizations the level width is essentially zero. The change in the statistics observed in small systems is due to a relatively small number of graphs with significant . Because the infinite system can be viewed as being composed of small ones, each of these parts having many neighbours, even a small probability to find a delocalized (finite width) level in a small system is sufficient for delocalization in the infinite system. This makes the typical decay rate in the infinite system much larger than the one in a collection of small ones. This explains why the crossover is always observed at a value of r n that is close to the one of Poisson statistics. To compute the critical value of the coupling constant expected in finite systems, we have evaluated the probability to find a level width in the solution of cavity equations for systems of a given size. The result is shown in Fig. 5 for a typical value of ɛ and . The crossing point observed by direct numerical diagonalization is expected to be found when the probability becomes non-zero. To avoid problems of numerical errors, we used the condition with δ 0 =0.004–0.02 and checked that the results are not sensitive to the specific value of δ 0 in this interval. Using this condition, we take into account both finite-size effects and we compute the finite-size corrections to the infinite-system ɛ c ( g ) predicted analytically. The final result for the apparent transition for small sizes is shown in Fig. 3 by the green line, it is shifted by a factor close to two with respect to the infinite-size ɛ c ( g ) shown by the red line. 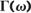Figure 5: Distribution function for a level width. The solution of cavity equations in finite random graphs gives a widely distributed widthof single spin-flip excitations. The inset shows the probability distribution offorω=0.35Win a random graph withN=20 spins and a coupling constantg=0.10. The right peak in this distribution corresponds to all graphs in which a significantis spontaneously formed. The main panel shows the weight of the graphs in which a significant(defined as) is formed as a function of the interaction constantg. The resulting value is only weakly sensitive to the value of the cut-offfor mostωandg. This allows us to determine the apparent critical value of the interaction constantg(ω) for the finite systems. The results are shown inFig. 3as a dashed line. Figure 5: Distribution function for a level width . The solution of cavity equations in finite random graphs gives a widely distributed width of single spin-flip excitations. The inset shows the probability distribution of for ω =0.35 W in a random graph with N =20 spins and a coupling constant g =0.10. The right peak in this distribution corresponds to all graphs in which a significant is spontaneously formed. The main panel shows the weight of the graphs in which a significant (defined as ) is formed as a function of the interaction constant g . The resulting value is only weakly sensitive to the value of the cut-off for most ω and g . This allows us to determine the apparent critical value of the interaction constant g(ω ) for the finite systems. The results are shown in Fig. 3 as a dashed line. Full size image Finally, when comparing the predictions of the cavity equations with the results of the exact diagonalization, we have to take into account that high-energy levels of the whole system correspond to many spin flips: the resulting decay rate is the sum of the decay rates of the individual flips. Because of the weak (logarithmic) dependence of the probability on this fact has a very weak effect on the expected transition. Because of the fast (exponential) dependence of the density of states on the energy, the typical spin flip contributing to the high energy level has a well-defined energy given by the saddle-point analysis presented in the Supplementary Information : . This allows us to map the energies, E , studied in the numerical diagonalization to a typical energy of a single flip, ɛ ( E ), and to compare the results of the numerical diagonalization and the solution of cavity equations as shown in Fig. 3 . How to cite this article: Cuevas, E. et al . Level statistics of disordered spin-1/2 systems and materials with localized Cooper pairs. Nat. Commun. 3:1128 doi: 10.1038/ncomms2115 (2012).